Fcp1-dependent dephosphorylation is required for M-phase-promoting factor inactivation at mitosis exit Correct execution of mitosis in eukaryotes relies on timely activation and inactivation of cyclin B-dependent kinase 1 (cdk1), the M-phase-promoting factor (MPF). Once activated, MPF is sustained until mitotic spindle assembly by phosphorylation-dependent feedback loops that prevent inhibitory phosphorylation of cdk1 and ubiquitin-dependent degradation of cyclin B. Whether subsequent MPF inactivation and anaphase onset require a specific phosphatase(s) to reverse these feedback loops is not known. Here we show through biochemical and genetic evidence that timely MPF inactivation requires activity of the essential RNA polymerase II-carboxy-terminal domain phosphatase Fcp1, in a transcription-independent manner. We identify Cdc20, a coactivator of the ubiquitin ligase anaphase-promoting complex/cyclosome (APC/C) required for cyclin degradation and anaphase onset, USP44, a deubiquitinating peptidase that opposes APC/C action, and Wee1, a cdk1 inhibitory kinase, as relevant Fcp1 targets. We propose that Fcp1 has a crucial role in the liaison between dephosphorylation and ubiquitination that drives mitosis exit. The establishment of mitosis requires phosphorylation of several substrates operated by several kinases [1] . Until mitotic spindle assembly, M-phase-promoting factor (MPF) activity itself is sustained through phosphorylation-dependent feedback loops [2] , [3] . Mitotic phosphorylations inhibit Wee1 and Myt1, cyclin B-dependent kinase 1 (cdk1) inhibitory kinases, activate Cdc25C, cdk1-activating phosphatase and implement the spindle assembly checkpoint (SAC), a safeguard mechanism that prevents premature cdk1 inactivation and anaphase onset by delaying degradation of cyclin B and of the anaphase inhibitor securin [2] , [3] , [4] , [5] , [6] , [7] , [8] , [9] . Although the precise mechanism(s) by which SAC requires phosphorylation is still unclear, it has been suggested that phosphorylation of Cdc20 and USP44 promotes SAC action [4] , [10] , [11] , [12] . To return to the interphase state, mitotic phosphorylations must be reversed by the end of mitosis. Indeed, it has been shown that, downstream of MPF inactivation, mitosis completion in vertebrate cells requires the action of phosphatases like PP1 and PP2A (refs 13 , 14 ). However, whether reversal of mitotic phosphorylations is required for MPF inactivation in vertebrates is unclear. In this study, by biochemical and genetic experiments in human cells, we show that at the end of mitosis timely MPF inactivation requires activity of the Fcp1 phosphatase. We identified Cdc20, Usp44 and Wee1 as crucial Fcp1 targets. We conclude that Fcp1 is required for mitosis exit by reversing phosphorylation of controllers of both proteolysis- and phosphorylation-dependent means of MPF inactivation. Fcp1 is required for M-phase exit in HeLa cell extracts To determine whether cdk1 inactivation and anaphase onset required reversal of MPF-sustaining phosphorylations, we first analysed the effect of the potent PP1 and PP2A phosphatases inhibitor okadaic acid (o.a.) on cyclin B degradation in HeLa cells. The cells were exiting mitosis on release from SAC-dependent arrest induced by the reversible microtubule inhibitor nocodazole. O.a. did not prevent cyclin B degradation and anaphase onset nor dissociation of the inhibitory SAC protein Mad2 from anaphase-promoting complex/cyclosome (APC/C). However, it substantially delayed dephosphorylation of several mitotic phosphoepitopes, recognized by the MPM-2 monoclonal antibody, and mitosis exit downstream cdk1 inactivation ( Supplementary Fig. S1 ), in agreement with previously described results [13] . Under our conditions, o.a. may robustly inhibit PP2A but only partly PP1, nevertheless, it has been shown that specific PP1 inhibition in checkpoint HeLa cell extracts did not prevent cdk1 inactivation [14] . Thus, if dephosphorylations were needed for cdk1 inactivation at mitosis exit they likely involved phosphatase(s) other than PP1 and PP2A. In the search for a relevant phosphatase(s), we considered recent genetic data from Aspergillus nidulans (AN) showing an antagonism between the essential, o.a. resistant, RNA polymerase II-carboxy-terminal domain phosphatase Fcp1 and cdk1 (ref. 15 ). In AN, a defective Fcp1 allele genetically interacted with an inhibitory phosphorylation-resistant cdk1 allele and forced expression of both alleles deranged mitosis and impaired nuclear separation [15] . However, as Fcp1 is a crucial transcription regulator, the genetic approach could not discern whether mitotic defects were due to lack of Fcp1-dependent dephosphorylation of mitotic regulators or rather to changes in gene expression [15] , [16] , [17] . To unveil a direct link between Fcp1 phosphatase activity and cdk1 inactivation, extracts from mitotic, SAC-arrested, HeLa cells were used that, devoid of nuclei, inactivate SAC, degrade cyclin B and progress out of M-phase in vitro (checkpoint extracts [18] ). Checkpoint extracts were either mock- or Fcp1-depleted, and Fcp1-depleted extracts were also reconstituted with recombinant, active, 3XFlag-tagged Fcp1 (3F-Fcp1; Supplementary Fig. S2 ) [17] . Whereas in control extracts, cyclin degradation was initiated after a 120-min lag and extracts exited the mitotic state thereafter, as indicated by decline in MPM-2 signal in Fcp1-depleted extracts cyclin B and MPM-2 signals remained stable for up to 6 h of incubation ( Fig. 1a ). Importantly, cyclin degradation and M-phase exit were restored in 3F-Fcp1-reconstituted extracts ( Fig. 1a ). Moreover, in undepleted extracts, a threefold excess of 3F-Fcp1 accelerated cyclin degradation and M-phase exit relatively to a control extract ( Fig. 1b ). The same excess of a mutant, catalytic inactive, Fcp1 version (3F-Fcp1-CD) on the contrary delayed both events ( Fig. 1b ). 3F-Fcp1-CD acted in a dominant negative manner perhaps by interacting with endogenous Fcp1 (see Supplementary Fig. S3 ). Thus, Fcp1 appears to be required for M-phase exit independently of its transcriptional role, perhaps by directly dephosphorylating crucial mitotic substrates. 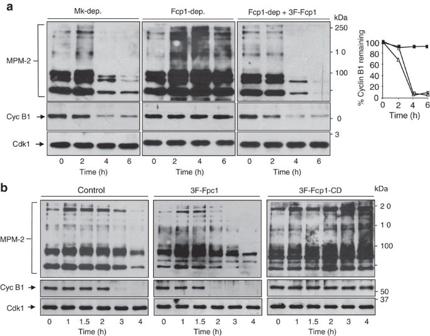Figure 1: Role for FCP1 in checkpoint extracts M-phase exit. (a) HeLa checkpoint extracts were mock-depleted (Mk-dep.), Fcp1-depleted (Fcp1-dep.) and a portion of Fcp1-depleted extract was reconstituted by adding back recombinant 3XFlag-tagged Fcp1 (Fcp1-dep.+3F-Fcp1). Samples were taken at the indicated time of incubation at 23 °C. Samples were probed for the indicated antigens, the MPM-2 antibody recognizes mitotic phosphoepitopes. The graph shows the percent (densitometric quantitation) of cyclin B1 remaining from time 0 of incubation in (open square) Mk-dep., (filled square) Fcp1-dep. and (open triangle) Fcp1-dep.+3F-Fcp1 extracts. (b) Checkpoint extract aliquots were incubated with buffer (control), or with a threefold excess of recombinant wild-type (3F-Fcp1) or catalytic inactive (3F-Fcp1-CD) Fcp1. Samples taken at the indicated time of incubation were separated on SDS–PAGE and blots probed for the indicated antigens. The data shown are representative of at least six independent experiments. Figure 1: Role for FCP1 in checkpoint extracts M-phase exit. ( a ) HeLa checkpoint extracts were mock-depleted (Mk-dep. ), Fcp1-depleted (Fcp1-dep.) and a portion of Fcp1-depleted extract was reconstituted by adding back recombinant 3XFlag-tagged Fcp1 (Fcp1-dep.+3F-Fcp1). Samples were taken at the indicated time of incubation at 23 °C. Samples were probed for the indicated antigens, the MPM-2 antibody recognizes mitotic phosphoepitopes. The graph shows the percent (densitometric quantitation) of cyclin B1 remaining from time 0 of incubation in (open square) Mk-dep., (filled square) Fcp1-dep. and (open triangle) Fcp1-dep.+3F-Fcp1 extracts. ( b ) Checkpoint extract aliquots were incubated with buffer (control), or with a threefold excess of recombinant wild-type (3F-Fcp1) or catalytic inactive (3F-Fcp1-CD) Fcp1. Samples taken at the indicated time of incubation were separated on SDS–PAGE and blots probed for the indicated antigens. The data shown are representative of at least six independent experiments. Full size image Fcp1-dependent dephosphorylations at M-phase exit To identify potential Fcp1 targets for MPF inactivation, we first analysed the dephosphorylation kinetics of proteins whose mitotic phosphorylation has been involved in the control of MPF activity during early stages of mitosis exit in cells. We analysed Wee1, Myt1 and Cdc25C, controllers of inhibitory cdk1 phosphorylation, and Cdc20, Cdc27, an APC/C member, and USP44, controllers of cyclin degradation, from HeLa cells sampled at short intervals during release from SAC-dependent arrest. Dephosphorylation was monitored by detecting increased protein mobility on SDS–polyacrylamide gel electrophoresis (PAGE) for all proteins and for Wee1, Myt1, Cdc25C and Cdc27 also by loss of site-specific mitotic phosphorylation. We developed an antibody recognizing phosphothreonine 239 of Wee1 (p-T239-Wee1), a crucial phosphorylation for cdk1-dependent inhibition of Wee1 [5] , [8] , whereas p-S83-Myt1, p-T48-Cdc25C and p-T244-Cdc27 were detected by commercially available antibodies ( Fig. 2a ). USP44 dephosphorylation was followed in cells transiently transfected with a V5-tagged USP44 expression vector ( Supplementary Fig. S4 ). Increased migration of Wee1, USP44, Cdc20 and loss of p-T239-Wee1 signal ensued rapidly after release from nocodazole, when cyclin B1 was still stable (by 10–20 min; Fig. 2a,b ). This was ahead of dephosphorylation of Myt1, Cdc25C and Cdc27, that begun at later time points, along with, or slightly after, initiation of cyclin B1 degradation (by 30–40 min; Fig. 2a,c ). Rapid p-T239-Wee1 dephosphorylation was also detected during SAC resolution in non-transformed human hTERT-RPE1 cells ( Supplementary Fig. S5 ). Thus, dephosphorylation of Wee1, Cdc20 and USP44 began concomitantly during spindle assembly and apparently before significant degradation of cyclin. Like the major biochemical reactions of mitosis exit in living cells, checkpoint extracts reproduced the changes in the phosphorylation status of these proteins during M-phase exit (see below), thus, we asked whether these changes depended on the presence of Fcp1. Indeed, depletion/reconstitution experiments showed that dephosphorylation of Wee1, particularly T239-Wee1, Cdc20 and USP44 depended on Fcp1 ( Fig. 3a ). Moreover, activities of Wee1 and USP44 were also dependent on the presence of Fcp1 ( Fig. 3b,c ). Wee1 kinase activity remained low in Fcp1-depleted extracts while it increased in control extracts and in Fcp1-reconstituted extract that exited M-phase ( Fig. 3b ). Ubiquitin peptidase activity of USP44, measured by an in vitro deubiquitination assay [10] , decreased during incubation in control and Fcp1-reconstituted extracts, which cycled from M-phase into interphase, whereas it remained high in Fcp1-depleted extract for the duration of the experiment ( Fig. 3c ). USP44 activity has been shown to help to maintain the binding of the SAC inhibitory Mad2 to Cdc20 and to regulate Cdc20 ubiquitination [10] , [19] . Indeed, we found that more than 90% of Mad2 had dissociated from Cdc20 after a 4-h incubation in control and Fcp1-reconstituted extracts, whereas dissociation was prevented in the Fcp1-depleted extract ( Fig. 3d ). In addition, while in control and Fcp1-reconstituted extracts about 60–70% of Cdc20 was degraded during incubation, Cdc20 remained stable in the Fcp1-depleted extract ( Fig. 3d ), further suggesting a functional relationship between Fcp1 and USP44 (refs 10 , 19 ). We also found that a short treatment with a cdk1 inhibitor accelerated Wee1, Cdc20 and USP44 dephosphorylations in control extracts but it failed to do so in Fcp1-depleted extracts ( Fig. 3e ). Together, these data strongly suggest that Fcp1 is required for MPF inactivation by reversing crucial mitotic phosphorylations and indicate a direct antagonism between Fcp1 and cdk1. 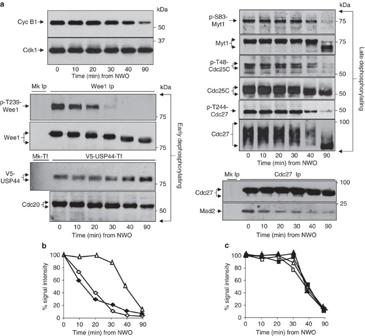Figure 2: Reversal of protein phosphorylation during mitosis exit. (a) SAC-arrested HeLa cells were released from arrest (nocodazole wash out; NWO) and sampled at indicated incubation time points. Indicated antigens were probed on total sample blots except p-T239-Wee1 and Wee1, probed on blots of Wee1 immunoprecipitates (Ips). Cdc27 and Mad2 were also probed on blots of Cdc27 Ips. All antigens were analyzed from samples of the same cell lysates except V5-tagged USP44, analysed by probing with an anti-V5 antibody lysates from HeLa cells previously transfected with a V5-tagged USP44 expression vector (V5-USP44-Tf; Mk-Tf=mock-transfected cells). (b) Densitometric quantification of signals from the immunoblots shown ina, expressed as percent of the time 0 value: (open triangles) Cyclin B1, (open diamonds) p-T239-Wee1, (closed diamonds) Cdc27-bound Mad2. (c) Densitometric quantification of signals from the immunoblots shown ina, expressed as percent of the time 0 value: (open triangles) Cyclin B1, (closed triangles) p-T244-Cdc27, (open squares) p-T48-Cdc25C and (closed squares) p-S83-Myt1. The data shown are representative of four independent experiments. Figure 2: Reversal of protein phosphorylation during mitosis exit. ( a ) SAC-arrested HeLa cells were released from arrest (nocodazole wash out; NWO) and sampled at indicated incubation time points. Indicated antigens were probed on total sample blots except p-T239-Wee1 and Wee1, probed on blots of Wee1 immunoprecipitates (Ips). Cdc27 and Mad2 were also probed on blots of Cdc27 Ips. All antigens were analyzed from samples of the same cell lysates except V5-tagged USP44, analysed by probing with an anti-V5 antibody lysates from HeLa cells previously transfected with a V5-tagged USP44 expression vector (V5-USP44-Tf; Mk-Tf=mock-transfected cells). ( b ) Densitometric quantification of signals from the immunoblots shown in a , expressed as percent of the time 0 value: (open triangles) Cyclin B1, (open diamonds) p-T239-Wee1, (closed diamonds) Cdc27-bound Mad2. ( c ) Densitometric quantification of signals from the immunoblots shown in a , expressed as percent of the time 0 value: (open triangles) Cyclin B1, (closed triangles) p-T244-Cdc27, (open squares) p-T48-Cdc25C and (closed squares) p-S83-Myt1. The data shown are representative of four independent experiments. 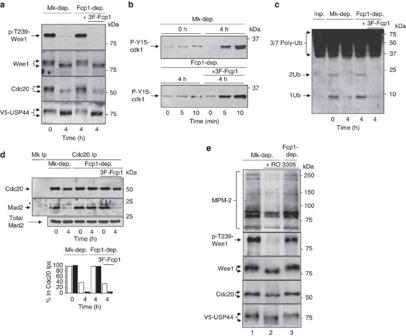Figure 3: Fcp1-dependent dephosphorylations in checkpoint extracts. Checkpoint extracts were mock-depleted (Mk-dep.), Fcp1-depleted (Fcp1-dep.) and 3F-Fcp1-reconstituted as inFig. 1a. At indicated time of incubation, (a) p-T239-Wee1 and Wee1 were probed on Wee1 immunoprecipitates (Ips), while Cdc20 on total samples. USP44 was analysed by mixing extracts with V5-USP44, immunopurified from transfected, SAC-arrested, cells before starting incubation and probing samples for V5 epitope. (b) Wee1 activity was assayed by mixing 3XFlag-tagged Wee1, immunopurified from transfected, SAC-arrested, cells with mock-depleted extract aliquots taken at time 0 and after a 4-h incubation at 23 °C and with Fcp1-depleted and 3F-Fcp1-reconstituted extracts taken after a 4-h incubation at 23 °C. After further 30 min incubation, kinase activity of reisolated Wee1 was assayedin vitrousing recombinant, catalytic dead, cyclin B-cdk1(KR) complex as substrate. Samples taken at 0, 5 and 10 min of kinase reaction were probed with an anti-p-Y15-cdk1 antibody. (c) USP44 activity was assayed by mixing V5-USP44, immunopurified from transfected, SAC-arrested, cells with mock-depleted extract aliquots taken at time 0 and after a 4-h incubation at 23 °C and with Fcp1-depleted and 3F-Fcp1-reconstituted extracts taken after a 4-h incubation at 23 °C. After further 30 min incubation, deubiquitinating activity of reisolated V5-USP44 was assayedin vitroon polyubiquitin chains (3/7 Poly-Ub) as substrate. The reactions were probed with an anti-ubiquitin antibody, the positions of the mono-, di- and poly-ubiquitin forms are indicated. (d) Cdc20 and Mad2 were probed on Cdc20 Ips taken from mock-depleted, Fcp1-depleted and 3F-Fcp1-reconstituted samples taken at indicated incubation times (asterisk, Ig). Mad2 was also probed in total extract samples (Total Mad2). The bar graph shows the level of (open bar) Cdc20 and (closed bar) Mad2 in Cdc20 Ips expressed as percent of time 0 sample values. (e) Mock-depleted extracts were incubated for 30 min at 23 °C minus (lane 1) or plus (lane 2) the cdk1 inhibitor RO 3306, along with Fcp1-depleted extract plus RO 3306 (lane 3). MPM-2 was probed from total samples, other antigens analysed as described ina. The data shown are representative of three independent experiments. Full size image Figure 3: Fcp1-dependent dephosphorylations in checkpoint extracts. Checkpoint extracts were mock-depleted (Mk-dep. ), Fcp1-depleted (Fcp1-dep.) and 3F-Fcp1-reconstituted as in Fig. 1a . At indicated time of incubation, ( a ) p-T239-Wee1 and Wee1 were probed on Wee1 immunoprecipitates (Ips), while Cdc20 on total samples. USP44 was analysed by mixing extracts with V5-USP44, immunopurified from transfected, SAC-arrested, cells before starting incubation and probing samples for V5 epitope. ( b ) Wee1 activity was assayed by mixing 3XFlag-tagged Wee1, immunopurified from transfected, SAC-arrested, cells with mock-depleted extract aliquots taken at time 0 and after a 4-h incubation at 23 °C and with Fcp1-depleted and 3F-Fcp1-reconstituted extracts taken after a 4-h incubation at 23 °C. After further 30 min incubation, kinase activity of reisolated Wee1 was assayed in vitro using recombinant, catalytic dead, cyclin B-cdk1(KR) complex as substrate. Samples taken at 0, 5 and 10 min of kinase reaction were probed with an anti-p-Y15-cdk1 antibody. ( c ) USP44 activity was assayed by mixing V5-USP44, immunopurified from transfected, SAC-arrested, cells with mock-depleted extract aliquots taken at time 0 and after a 4-h incubation at 23 °C and with Fcp1-depleted and 3F-Fcp1-reconstituted extracts taken after a 4-h incubation at 23 °C. After further 30 min incubation, deubiquitinating activity of reisolated V5-USP44 was assayed in vitro on polyubiquitin chains (3/7 Poly-Ub) as substrate. The reactions were probed with an anti-ubiquitin antibody, the positions of the mono-, di- and poly-ubiquitin forms are indicated. ( d ) Cdc20 and Mad2 were probed on Cdc20 Ips taken from mock-depleted, Fcp1-depleted and 3F-Fcp1-reconstituted samples taken at indicated incubation times (asterisk, Ig). Mad2 was also probed in total extract samples (Total Mad2). The bar graph shows the level of (open bar) Cdc20 and (closed bar) Mad2 in Cdc20 Ips expressed as percent of time 0 sample values. ( e ) Mock-depleted extracts were incubated for 30 min at 23 °C minus (lane 1) or plus (lane 2) the cdk1 inhibitor RO 3306, along with Fcp1-depleted extract plus RO 3306 (lane 3). MPM-2 was probed from total samples, other antigens analysed as described in a . The data shown are representative of three independent experiments. Full size image Putative direct Fcp1 targets for M-phase exit We asked whether Fcp1 could directly dephosphorylate the relevant substrates for exit from mitosis. In vitro , active 3F-Fcp1 dephosphorylated mitotic Wee1, Cdc20 and USP44 but not Cdc27 ( Fig. 4a,b ). When analysed by SDS–PAGE, 3F-Fcp1-dephosphorylated proteins had an intermediate migration between that from SAC-arrested and G1 cells ( Fig. 4a ), indicating that Fcp1 dephosphorylated only a subset of phosphosites in these proteins, perhaps favouring the action of other phosphatases [1] , [14] , [15] . Several reports have demonstrated the relevance for mitotic phosphoryation of Cdc20 and Wee1, particularly p-T239-Wee1, in the control of their activies towards MPF [5] , [7] , [8] , [11] , [12] . USP44 activity has also been hypothesized to be regulated by phosphorylation, in particular, mitotic phosphorylation is thought to stimulate its deubiquitinating activity required to sustain SAC [10] . We found that pretreatment of active USP44 in vitro , isolated from SAC-arrested cells, with active 3F-Fcp1 substantially reduced USP44 ubiquitin peptidase activity, whereas pretreatment with the catalytic dead 3F-Fcp1-CD mutant had little effect ( Fig. 4c ). In addition, we produced a mutant human USP44 (USP44-4A) protein that cannot be phosphorylated at four potential cdk1 or mitotic sites (ser-169, -239, -401 and threo-269). When expressed and analysed in SAC-arrested cells, USP44-4A showed a faster migration on SDS–PAGE than wild-type USP44, suggesting that these residues are phosphorylated under active SAC conditions in cells ( Fig. 4d ). In addition, when assayed in vitro , USP44-4A had significantly reduced ubiquitin peptidase activity compared with wild-type USP44 ( Fig. 4e ). These findings provide a mechanistic explanation for how Fcp1 activity could promote exit from mitosis and suggest that Fcp1 may directly promote crucial dephosphorylations that are required for MPF inactivation. 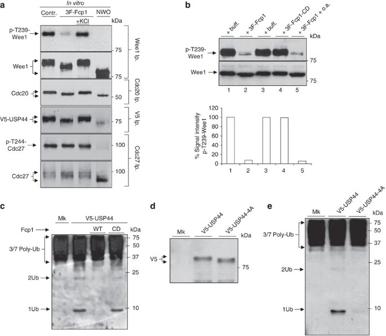Figure 4: Putative direct Fcp1 substrates for M-phase exit. (a) Wee1, Cdc20 and Cdc27 were immunoprecipitated (Ip) from nocodazole-arrested HeLa cell samples and from cell samples taken after 120 min incubation from nocodazole wash out (NWO). USP44 was immunopurified from previously V5-USP44-transfected HeLa cells under analogous conditions. Ips from nocodazole-arrested cells were divided into three samples and incubated for 30 min at 23 °C with buffer, as control (Contr.), or with active recombinant 3F-Fcp1 in the absence (3F-Fcp1) or in the presence of 120 mM KCl (3F-Fcp1+KCl), a salt that inhibits Fcp1 catalytic activity30. After incubation, the Ips were resolved, along with those from NWO cells, on SDS–PAGE and blots probed for the indicated antigens. (b) Wee1 was Ip from nocodazole-arrested HeLa cells. The Ip was split into five samples and incubated (lane 1) with Fcp1 phosphatase buffer, (lane 2) buffer+active 3F-Fcp1, (lane 3) buffer, (lane 4) buffer+inactive 3F-Fcp1-CD and (lane 5) buffer+active 3F-Fcp1+okadaic acid (o.a., 100 nM, a concentration shown to inhibit both PP2A and PP1 catalytic activitiesin vitro31. After incubation, samples were split in two, resolved on parallel SDS–PAGE and blots probed for the indicated antigens. The bar graph shows densitometric quantification of the p-T239-Wee1 signal expressed as normalized percent of the value from control sample in lane 1. The data shown are representative of at least three independent experiments. (c) V5 Ips were performed from mock- (Mk) and V5-USP44-transfected (V5-USP44), nocodazole-arrested, HeLa cell lysates. The V5 Ip from V5-USP44-transfected cells was split into three portions and incubated with either buffer, recombinant 3F-Fcp1 or inactive 3F-Fcp1-CD for 30 min at 23 °C. V5-USP44 was reisolated and its deubiquitinating activity assayedin vitroas previously described, the positions of the mono-, di- and poly-ubiquitin (Poly-Ub) forms are indicated. (d) An anti-V5 blot from samples of Mk, wild-type (WT) V5-USP44- and mutant V5-USP44-4A-transfected SAC-arrested HeLa cells. (e) Deubiquitinating activity of wild-type V5-USP44 and mutant V5-USP44-4A, isolated from SAC-arrested HeLa cells. Figure 4: Putative direct Fcp1 substrates for M-phase exit. ( a ) Wee1, Cdc20 and Cdc27 were immunoprecipitated (Ip) from nocodazole-arrested HeLa cell samples and from cell samples taken after 120 min incubation from nocodazole wash out (NWO). USP44 was immunopurified from previously V5-USP44-transfected HeLa cells under analogous conditions. Ips from nocodazole-arrested cells were divided into three samples and incubated for 30 min at 23 °C with buffer, as control (Contr. ), or with active recombinant 3F-Fcp1 in the absence (3F-Fcp1) or in the presence of 120 mM KCl (3F-Fcp1+KCl), a salt that inhibits Fcp1 catalytic activity [30] . After incubation, the Ips were resolved, along with those from NWO cells, on SDS–PAGE and blots probed for the indicated antigens. ( b ) Wee1 was Ip from nocodazole-arrested HeLa cells. The Ip was split into five samples and incubated (lane 1) with Fcp1 phosphatase buffer, (lane 2) buffer+active 3F-Fcp1, (lane 3) buffer, (lane 4) buffer+inactive 3F-Fcp1-CD and (lane 5) buffer+active 3F-Fcp1+okadaic acid (o.a., 100 nM, a concentration shown to inhibit both PP2A and PP1 catalytic activities in vitro [31] . After incubation, samples were split in two, resolved on parallel SDS–PAGE and blots probed for the indicated antigens. The bar graph shows densitometric quantification of the p-T239-Wee1 signal expressed as normalized percent of the value from control sample in lane 1. The data shown are representative of at least three independent experiments. ( c ) V5 Ips were performed from mock- (Mk) and V5-USP44-transfected (V5-USP44), nocodazole-arrested, HeLa cell lysates. The V5 Ip from V5-USP44-transfected cells was split into three portions and incubated with either buffer, recombinant 3F-Fcp1 or inactive 3F-Fcp1-CD for 30 min at 23 °C. V5-USP44 was reisolated and its deubiquitinating activity assayed in vitro as previously described, the positions of the mono-, di- and poly-ubiquitin (Poly-Ub) forms are indicated. ( d ) An anti-V5 blot from samples of Mk, wild-type (WT) V5-USP44- and mutant V5-USP44-4A-transfected SAC-arrested HeLa cells. ( e ) Deubiquitinating activity of wild-type V5-USP44 and mutant V5-USP44-4A, isolated from SAC-arrested HeLa cells. Full size image Fcp1 affects mitotis exit in human cells Having established that Fcp1 phosphatase activity is required for MPF inactivation independently of its effects on transcription regulation in the in vitro checkpoint extract system, we asked whether Fcp1 affected SAC resolution and mitosis exit in living cells. Strong Fcp1 downregulation could be obtained in HeLa cells by treatment with a pool of small interfering RNA (siRNA) targeting the Fcp1-coding region ( Fig. 5a ) or with one siRNA targeting a segment of the Fcp1 3′ untranslated region (UTR; Fig. 5b ). Strong Fcp1 downregulation delayed cell cycle progression at different cell cycle stages, however, Fcp1-siRNA-treated cells that could be SAC-arrested, following nocodazole treatment, were substantially delayed in cyclin B1 degradation and mitosis exit upon release from SAC-arrest ( Fig. 5a ). Although we cannot exclude subtle alterations in spindle assembly, morphological analysis indicated that Fcp1-siRNA-treated cells progressed into metaphase with similar kinetics as control cells but were delayed thereafter. In Fcp1-siRNA-UTR-treated cells, the mitosis exit delay was reversed by re-expression of siRNA-resistant 3F-Fcp1 ( Fig. 5b,c ). We asked whether overexpression of 3F-Fcp1 or the catalytically dead 3F-Fcp1-CD mutant would affect mitosis exit in HeLa cells similar to what was observed in checkpoint extracts. Indeed, HeLa cells overexpressing 3F-Fcp1, about threefold over endogenous Fcp1 levels, showed an acceleration in exiting mitosis upon SAC resolution while expression of the same level of 3F-Fcp1-CD significantly delayed mitosis exit kinetics upon SAC resolution ( Fig. 5d,e ). These data confirm the requirement for Fcp1 in SAC-dependent arrest resolution in living cells. Although Fcp1 overexpressing cells tended to adapt and exit mitosis inspite of an impaired spindle assembly, relatively faster than control cells upon prolonged incubation in nocodazole, they were efficiently SAC-arrested after a 14-h nocodazole treatment. In Fcp1 overexpressing cells, adaptation was significantly accelerated when SAC was induced by taxol, a microtubule poison that affects spindle assembly by impairing microtubule depolymerization rather than polymerization like nocodazole ( Fig. 5f ). That Fcp1-overexpressing cells adapted more rapidly under taxol rather than nocodazole may reflect the fact that either the two poisons have different potency in stimulating SAC, for instance in activating SAC effector proteins, or that Fcp1 action may be favoured by structural requirements including kinetochore-spindle pole microtubule-mediated connection, that form in rudimental spindles under taxol rather than nocodazole regimen. That Fcp1 was required to reverse the inhibitory effects of an activated SAC on MPF inactivation was also indicated by the finding that Fcp1-siRNA-treated cells were resistant to the SAC override induced by reversine, an inhibitor of the SAC kinase Mps1 (ref. 20 ; Fig. 5g ). 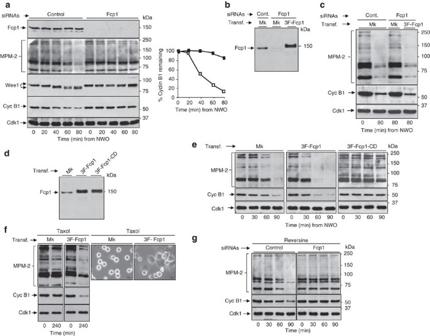Figure 5: Fcp1 affects mitosis exit in cells. (a) 72 h post-transfection, control (Cont.), non-targeting, or Fcp-1-targeting (coding region), siRNAs-transfected HeLa cells were treated with nocodazole for 14 h. SAC-arrested cells were washed free of nocodazole (NWO) and sampled at indicated time points during incubation in fresh medium. Cell lysates were directly probed for indicated antigens. The graph shows a densitometric quantification of cyclin B1 signal remaining, expressed as percent of time 0 value, in (open squares) control cells and (filled squares) Fcp-1-targeted cells. (b,c) HeLa cells were treated with non-targeting siRNA or with a siRNA-targeting Fcp1 3′UTR. After 40 h, cells were transfected with either mock- (Mk-) or 3F-Fcp1-expressing vectors. 32 h later cells were treated with nocodazole for 14 h. SAC-arrested cells were either (b) harvested and probed for Fcp1 on total samples or (c) washed free of nocodazole (NWO), sampled at indicated time points during incubation in fresh medium, and probed for indicated antigens. (d,e) HeLa cells were transfected (transf.) with either Mk-, 3F-Fcp1- or 3F-Fcp1-CD-expressing vectors before nocodazole treatment. SAC-arrested cells were either (d) harvested and probed for Fcp1 on total samples or (e) washed free of nocodazole (NWO), sampled at indicated time points during incubation in fresh medium and probed for indicated antigens. (f) SAC-arrested Mk- or 3F-Fcp1-transfected HeLa cells were collected and released from nocodazole into fresh medium containing taxol. After further 240 min incubation, cells were either sampled and lysates probed for indicated antigens (left panels) or photographed in light microscopy (right panels). During 240 min incubation with taxol, about 10% Mk-transfected and 70% 3F-Fcp1-transfected cells exited mitosis and reattached to the culture dish. Scale bars, 10 μm. (g) Control, non-targeting or Fcp-1-targeting, siRNAs-transfected HeLa cells were treated with nocodazole for 14 h. SAC-arrested cells were replated into new dishes and further incubated, always in the presence of nocodazole, following addition of the MPS1 inhibitor reversine. Total cell extract samples, taken at indicated time points from reversine addition, were probed for indicated antigens. The data shown are representative of three independent experiments. Figure 5: Fcp1 affects mitosis exit in cells. ( a ) 72 h post-transfection, control (Cont. ), non-targeting, or Fcp-1-targeting (coding region), siRNAs-transfected HeLa cells were treated with nocodazole for 14 h. SAC-arrested cells were washed free of nocodazole (NWO) and sampled at indicated time points during incubation in fresh medium. Cell lysates were directly probed for indicated antigens. The graph shows a densitometric quantification of cyclin B1 signal remaining, expressed as percent of time 0 value, in (open squares) control cells and (filled squares) Fcp-1-targeted cells. ( b , c ) HeLa cells were treated with non-targeting siRNA or with a siRNA-targeting Fcp1 3′UTR. After 40 h, cells were transfected with either mock- (Mk-) or 3F-Fcp1-expressing vectors. 32 h later cells were treated with nocodazole for 14 h. SAC-arrested cells were either ( b ) harvested and probed for Fcp1 on total samples or ( c ) washed free of nocodazole (NWO), sampled at indicated time points during incubation in fresh medium, and probed for indicated antigens. ( d , e ) HeLa cells were transfected (transf.) with either Mk-, 3F-Fcp1- or 3F-Fcp1-CD-expressing vectors before nocodazole treatment. SAC-arrested cells were either ( d ) harvested and probed for Fcp1 on total samples or ( e ) washed free of nocodazole (NWO), sampled at indicated time points during incubation in fresh medium and probed for indicated antigens. ( f ) SAC-arrested Mk- or 3F-Fcp1-transfected HeLa cells were collected and released from nocodazole into fresh medium containing taxol. After further 240 min incubation, cells were either sampled and lysates probed for indicated antigens (left panels) or photographed in light microscopy (right panels). During 240 min incubation with taxol, about 10% Mk-transfected and 70% 3F-Fcp1-transfected cells exited mitosis and reattached to the culture dish. Scale bars, 10 μm. ( g ) Control, non-targeting or Fcp-1-targeting, siRNAs-transfected HeLa cells were treated with nocodazole for 14 h. SAC-arrested cells were replated into new dishes and further incubated, always in the presence of nocodazole, following addition of the MPS1 inhibitor reversine. Total cell extract samples, taken at indicated time points from reversine addition, were probed for indicated antigens. The data shown are representative of three independent experiments. Full size image Requirements for Fcp1 action at mitosis exit Recent evidence has shown that SAC silencing requires APC/C-dependent ubiquitination and proteolysis, in a mutual antagonism between APC/C and SAC [10] , [21] , [22] . As previously described for Cdc20 dephosphorylation and Mad2 dissociation from the APC/C–Cdc20 complex [21] , we found that Wee1 and USP44 dephosphorylation was prevented when cells were released from nocodazole arrest into a proteasome inhibitor-containing medium ( Supplementary Fig. S6 ). In addition, by coimmunoprecipitation experiments Fcp1 was shown to transiently interacted with Cdc27 shortly after release from nocodazole arrest ( Fig. 6a ), and that p-T239-Wee1 dephosphorylation was prevented in cells depleted of Cdc27 by siRNAs, even after prolonged incubation following nocodazole release ( Fig. 6b ). Although lack of APC/C-dependent proteolysis may be rather indirectly required for Fcp1 action, our data suggest that the two functions are linked in a feedforward loop for exit from mitosis. Assays of total Fcp1 activity from cells before and after SAC resolution did not reveal significant changes ( Supplementary Fig. S7 ). Thus, either Fcp1 activity is constant and its substrate accessibility is regulated or activity of a small fraction of total Fcp1, localized at particular subcellular compartments, is regulated perhaps through an ubiquitination-proteolysis sensitive mechanism. Further work will be required to establish how Fcp1 action is precisely regulated. Nevertheless, in agreement with the idea that localized Fcp1 may be relevant for SAC inactivation and mitosis exit, recent observations indicated that Fcp1 localizes at centromeres in chromosomes isolated from mitotic cells [23] . Moreover, analysing Fcp1 localization by indirect immunofluorescence in fixed mitotic cells, we found that Fcp1 was detectable at centrosomes in prometaphase, at spindle and spindle poles in metaphase and at spindle midzone and midbody in anaphase and telophase-G1, respectively, thus, regulation of spindle localized Fcp1 activity might be crucial for mitosis exit ( Fig. 6c ). In addition, Fcp1 localization also suggests that the phosphatase might have further roles in anaphase and cytokinesis. Some APC/C members have been shown to localize at spindle poles and at unattached kinetochores, where they could be bound to inhibitory SAC proteins [24] , whereas some SAC proteins have been show to relocalize from kinetochores to spindle poles upon bi-orientation [4] , [25] . Fcp1 might be activated upon spindle assembly at spindle poles where, in turn, it may act to silence the SAC. 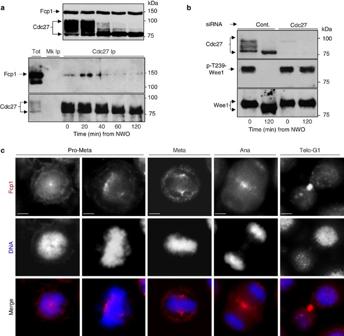Figure 6: Requirements for Fcp1 activity. (a) SAC-arrested HeLa cells were released from arrest (nocodazole wash out; NWO) and sampled at indicated incubation time points. Top panel: Fcp1 and Cdc27 were probed on total extract samples. Bottom panel: Fcp1 and Cdc27 were probed on blots of Cdc27 Ips. (b) 48 h post-transfection, control (Cont.), non-targeting, or Cdc27-targeting siRNAs-transfected HeLa cells were treated with nocodazole for 14 h. SAC-arrested cells, that detached from the substrate, were released from arrest (nocodazole wash out; NWO), sampled at indicated incubation time points and lysates were directly probed for Cdc27, whereas p-T239-Wee1 and total Wee1 were probed on blots of Wee1 Ips. (c) Indirect fluorescence immunostaining of Fcp1 (red), and chromatin (blue) staining, of HeLa cells at the indicated mitotic stages. Scale bars, 5 μm. Figure 6: Requirements for Fcp1 activity. ( a ) SAC-arrested HeLa cells were released from arrest (nocodazole wash out; NWO) and sampled at indicated incubation time points. Top panel: Fcp1 and Cdc27 were probed on total extract samples. Bottom panel: Fcp1 and Cdc27 were probed on blots of Cdc27 Ips. ( b ) 48 h post-transfection, control (Cont. ), non-targeting, or Cdc27-targeting siRNAs-transfected HeLa cells were treated with nocodazole for 14 h. SAC-arrested cells, that detached from the substrate, were released from arrest (nocodazole wash out; NWO), sampled at indicated incubation time points and lysates were directly probed for Cdc27, whereas p-T239-Wee1 and total Wee1 were probed on blots of Wee1 Ips. ( c ) Indirect fluorescence immunostaining of Fcp1 (red), and chromatin (blue) staining, of HeLa cells at the indicated mitotic stages. Scale bars, 5 μm. Full size image Together our data demonstrate a crucial role for Fcp1 phosphatase in the exit from mitosis. By targeting Cdc20 and USP44, Fcp1 appears to be required to reverse SAC-sustaining phosphorylations. At the same time, by targeting the cdk1 inhibitory kinase Wee1, Fcp1 reverses phosphorylation-dependent means of cdk1 inhibition, suggesting that, like in embryonic systems, this mechanism is an integral component of the somatic cell mitosis exit programme [9] . Indeed, our preliminary data indicate that inhibitory phosphorylation of cdk1 affects cyclin degradation and correct anaphase execution in somatic human cells as well (RDM, LP, AP, RV and DG, unpublished results). Downstream cdk1 inactivation, PP1 and PP2A appear to be required for mitosis completion in vertebrates [13] , [14] . Thus, these phosphatases are likely to take the upper hand and complete mitosis exit once cdk1 inactivation has begun in a Fcp1-dependent manner. Nevertheless, it is possible that Fcp1 action may begin cdk1 inactivation and, at the same time, promote the action of other phosphatase. In this regard, it will be interesting to investigate a possible relationship between Fcp1 and Greatwall kinase, a major kinase controlling PP2A activity in mitosis [26] , [27] . Although we do not know the precise mechanisms that regulate Fcp1 activity at M-phase exit, our data suggest that Fcp1 promotes SAC resolution by helping the SAC-silencing capacity of APC/C and reducing localized cdk1 activity [4] , [9] , [11] , [23] , [24] , [25] , [28] . During spindle assembly, an activatory relationship between APC/C and Fcp1 keeps resolving binding of activated SAC proteins to APC/C Cdc20 ; however, SAC proteins are continuously activated and reloaded onto APC/C Cdc20 at unattached kinetochores. As chromosome attachment and bi-orientation proceeds SAC robustness weakens. This way, cdk1 inactivation and anaphase onset ensues once SAC proteins activation has dropped to a minimum upon bi-orientation of the last replicated chromosome. As Fcp1 also resets RNAP II at the end of mitosis to allow transcription resumption in daughter cells [16] , [29] , [30] , our data suggest that the phosphatase has a crucial role in coordinating cell division with gene transcription. Checkpoint extracts preparation To prepare checkpoint extracts, HeLa cells arrested at the G1-S boundary by a double thymidine (2 mM) block were released into nocodazole (100 ng ml −1 ) for 11 h. Detached cell were washed once with ice-cold PBS and lysed in 75% pellet volume with extraction buffer (20 mM HEPES, pH 7.6, 5 mM KCl, 1 mM dithiothreitol) by three freeze–thaw cycles. Lysate was centrifuged at 16,000 g for 1 h at 4 °C and supernatant stored in small aliquots at −80 °C after addition of 5 mM MgCl 2 and 10% glycerol. On thawing, extracts were supplemented with a 20× energy regeneration mix (to give final concentration of 1 mM ATP, 10 mM phosphocreatine and 0.1 mg ml −1 creatine phosphokinase) before incubation at 23 °C. For immunodepletion experiments, energy regeneration mix was added after the immunodepletion procedure, just before incubation. Where indicated, RO 3306 was added at 10 μM. Cell culture and recombinant protein production HeLa and human embryonic kidney (HEK) 293 T cells were grown and treated as described [21] . HTERT-RPE1 cells were grown in DMEM/F12+10% fetal bovine serum. Nocodazole was used at 100 nM, taxol at 1 μM, o.a. at 1 μM (Calbiochem). Expression vector transfections were performed with FuGENE 6 (Roche), according to the manufacturer's specifications. V5-USP44 expression vector was obtained by transferring pENTR221-USP44 clone into V5-tagged pcDNA3.1 vector (Invitrogen). To generate the USP44-4A mutant, ser-169, -239, -401 and threo-269 of human USP44 were mutagenized into alanine (5′-GGTAAAATCTTTCGAACATGGTTTGAACAAGCACCCATTGGAAGAAA-3′; 5′-CAGCACAAACGCCAGCAGCACCAGCAAAAGATAAA-3′; 5′-GAAAGTGGGCGTTGGTCGCACCATTTGCTATGCTA-3′; 5′-TCAGTTAAACGAAGGCCAATAGTAGCTCCTGGTGTAAC-3′) by QuikChange II XL-sitedirected mutagenesis kit (Agilent Technologies) using the V5-tagged pcDNA3.1 USP44 vector as template. For siRNAs experiments, HeLa cells were transfected with ON-TARGET plus SMARTpool targeting Cdc27 and Fcp1 (coding region) and with ON-TARGETplus non-targeting pool as a control (Thermo Scientific Dharmacon). The siRNA targeting the 3′UTR of human Fcp1 (5′-GUAAGUGACAGGUGUUAAA-3′) was purchased from Dharmacon. Downregulation by more than 90% of the proteins was obtained after a 48-h transfection for Cdc27, and after a 72-h transfection for Fcp1. To generate the Fcp1 catalytic inactive version, aspartic acid residue 188 of human Fcp1, the first aspartic acid in the DxDxT/V catalytic signature [30] , was mutagenized into asparagine (5′-CTGGTGCTCATGGTGAACTTGGACCAGACGT-3′) by QuikChange II XL-site-directed mutagenesis kit using the 3XFlag-Fcp1 expression construct [17] as template. 3XFlag-tagged Fcp1 proteins were prepared from HEK-293 T 72-h post p3XFLAG-CMV-10-Fcp1 transfection [17] . Cell lysates were incubated with an anti-FLAG M2 affinity gel (Sigma) at 4 °C for 1 h. Beads were extensively washed with lysis buffer and extraction buffer (EXB; 20 mM HEPES, pH 7.6, 5 mM KCl, 1 mM dithiothreitol) and protein eluted in EXB+100 μg ml −1 3XFLAG peptide (Sigma). Recombinant Xenopus cyclin B and catalytic dead cdk1 (KR) mutant were a gift of Julian Gannon. Immunological procedures Anti-p-ser-83-Myt1, anti-Myt1, anti-p-thr-48-Cdc25C and anti-p-tyr-15-cdk1 antibodies were from Cell Signaling Technology. Anti-p-thr-244-Cdc27 antibody was from Novus Biologicals. Anti-MPM-2 antibody was from Millipore. Monoclonal anti-FLAG M2 and anti-V5 agarose-conjugate were from Sigma. Unconjugated anti-V5 antibody was from Invitrogen. Anti-Fcp1 antibodies were from Bethyl laboratories and Santa Cruz Biotechnology. Rabbit polyclonal antibodies against phosphothreonine 239 of human Wee1 were raised using PQVNINPF(p)TPDSLL peptide as immunogen; peptide synthesis, rabbit inoculation, serum production and cross-affinity antibody purification were carried out by Polypeptide Group. Other antibodies were from Santa Cruz Biotechnology. Immunofluorescence staining was performed as described [21] , using an anti-Fcp1 antibody from Santa Cruz Biotechnology. Immunoprecipitations and immunoblots were performed as described [21] . Densitometric quantifications of immunoblot signal intensity were performed by using the ImageJ software. For immunodepletion experiments, 20 μg of anti-Fcp1 Igs (10 μg, Santa Cruz Biotechnology+10 μg Bethyl) or 20 μg of nonimmune Igs, as control, were preadsorbed to protein A+G-agarose beads (20 μl of a 50% EXB/protein A+G-agarose beads) by rotation overnight at 4 °C. Checkpoint extracts were incubated with 1/10 volume packed pre-adsorbed beads on rotation for 90 min at 4 °C. Samples were spun at 16,000 g for 5 min at 4 °C and supernatants isolated. In reconstitution experiments, 40 ng μl −1 of recombinant 3F-Fcp1 was added back to Fcp1-depleted extracts (1/20 of extract volume); addition of same volume of elution buffer, without 3F-Fcp1, to Fcp1-depleted extracts had no effect. In vitro treatments and deubiquitination assay Substrates for in vitro dephosphorylation, immunoprecipitated from nocodazole-arrested HeLa cells, were washed in Fcp1 phosphatase assay buffer (FPAB; 20 mM HEPES, pH 7.6, 10 mM MgCl 2 , 1 mM dithiothreitol), mixed and incubated at 23 °C for 30 min in constant mixing with FPAB+1/10 volume of EXB+100 μg ml −1 FLAG peptide, as control, and with FPAB+1/10 volume of EXB+100 μg ml −1 3XFLAG peptide+eluted 3F-Fcp1 protein, plus or minus 120 mM KCl. For USP44 deubiquitination assay, and USP44 pretreatment with Fcp1, V5-USP44 immunoprecipitated from V5-USP44-transfected or mock-transfected, nocodazole-arrested HeLa cells, were washed once in FPAB and mixed with FPAB containing 1/10 volume of EXB+100 μg ml −1 FLAG peptide, as control, or FPAB containing 1/10 volume of EXB+100 μg ml −1 FLAG peptide+eluted 3F-Fcp1 protein. Following incubation at 23 °C for 30 min in constant mixing, beads were washed with deubiquitination buffer (25 mM Tris–HCl pH 7.5, 50 mM NaCl, 10 mM MgCl 2 , 2 mM dithiothreitol, 15 mM creatine phosphate, 2 mM ATP) and incubated again with polyubiquitin chains (Ub3-7, Boston Biochem) in deubiquitination buffer for 60 min at 30 °C in constant mixing. Supernatants, separated on 16% acrylamide SDS–PAGE, were probed with an anti-ubiquitin antibody. To assay USP44 from mock-depleted, Fcp1-depleted and Fcp1-reconstituted extracts, beads containing V5-USP44 immunoprecipitates from V5-USP44-transfected, nocodazole-arrested, HeLa cells were mixed with extracts aliquots taken at time 0 or after 4 h from start of incubation at 23 °C. V5-USP44 beads were incubated with extracts aliquots for further 30 min at 23 °C in constant shaking. V5-USP44 beads were reisolated and, then, washed and assayed for deubiquitination activity as described above. Wee1 activity was assayed by mixing 3XFlag-tagged Wee1, isolated from 3-F-Wee1 expression vector (a gift of Vincenzo D'Angiolella) -transfected and nocodazole-arrested HeLa cells, with extract aliquots taken either at time 0 or after a 4-h preincubation at 23 °C. After further 30 min incubation at 23 °C, Wee1 was reisolated and its kinase activity was assayed using recombinant, catalytic dead, cyclin B–cdk1(KR) complex as substrate during 0, 5 and 10 min of kinase reaction time. Samples were SDS–PAGE separated, blotted and probed with an anti-p-Y15-cdk1 antibody. How to cite this article: Visconti, R. et al . Fcp1-dependent dephosphorylation is required for M-phase-promoting factor inactivation at mitosis exit. Nat. Commun. 3:894 doi: 10.1038/ncomms1886 (2012).